Large resistivity modulation in mixed-phase metallic systems In numerous systems, giant physical responses have been discovered when two phases coexist; for example, near a phase transition. An intermetallic FeRh system undergoes a first-order antiferromagnetic to ferromagnetic transition above room temperature and shows two-phase coexistence near the transition. Here we have investigated the effect of an electric field to FeRh/PMN-PT heterostructures and report 8% change in the electrical resistivity of FeRh films. Such a ‘giant’ electroresistance (GER) response is striking in metallic systems, in which external electric fields are screened, and thus only weakly influence the carrier concentrations and mobilities. We show that our FeRh films comprise coexisting ferromagnetic and antiferromagnetic phases with different resistivities and the origin of the GER effect is the strain-mediated change in their relative proportions. The observed behaviour is reminiscent of colossal magnetoresistance in perovskite manganites and illustrates the role of mixed-phase coexistence in achieving large changes in physical properties with low-energy external perturbation. The past decades have witnessed dramatic discoveries in carrier-doped, strongly correlated complex oxides, typified by the emergence of high-temperature superconductivity in doped antiferromagnetic (AFM) cuprates and colossal magnetoresistance (CMR) in doped manganites [1] , [2] ; interestingly, reversible resistance switching induced by external electric fields on various manganites shows large electroresistance (ER) response and provides a great potential as an emerging non-volatile memory technology [3] , [4] , [5] , [6] . Although the detailed mechanism of high-temperature superconductivity remains to be understood, CMR effect in the manganites is known to result from coexisting and competing ferromagnetic (FM) metallic and AFM-insulating phases in the CMR regime [7] , [8] . An analogous response caused by mixed-phase coexistence in non-magnetic, uncorrelated oxides is found in the relaxor family of ferroelectrics, in which large dielectric and piezoelectric responses are observed near morphotropic phase boundaries [9] , [10] . In thin-film BiFeO 3 , epitaxial strain leads to the formation of a nanoscale, mixed-phase ensemble of two crystal structures that can be reversibly transformed between each other with electric fields, leading to large piezoelectric responses [11] , [12] . Although these examples (as a direct consequence of mixed-phase coexistence) all occur in systems that are insulating (at least until chemically doped), we extend the same concept to metallic systems of FeRh in this report. FeRh exhibits a temperature-dependent first-order phase transition at ~100 °C from an AFM (low temperature) to a FM (high temperature) phase that is characterized by 1% expansion in the volume [13] , [14] , [15] , [16] , [17] , [18] , [19] . Although the origin of the phase transition has long been a subject of theoretical studies [20] , [21] , it is now believed to result from different temperature dependencies of the entropy in the two phases [22] , [23] . The transition has recently been shown to persist in thin films [17] , [24] and the substrate dependence of the transition has been exploited in heterostructures of FeRh deposited on ferroelectric BaTiO 3 to induce the FM to AFM transition using an electric field [25] . We report large electric-field-induced changes in resistivity in a thin film of the intermetallic FeRh deposited on a piezoelectric substrate and demonstrate that the response results from the competition between coexisting AFM and FM phases with different resistivities. Growth and characterization We deposit FeRh films onto single crystals of [001]-oriented relaxor ferroelectric 0.72PbMg 1/3 Nb 2/3 O 3 –0.28PbTiO 3 (PMN-PT) [26] , [27] , [28] using both molecular-beam epitaxy (MBE) and ultra-high vacuum sputtering techniques. Details of the synthesis protocols used in our study, and both the structural and chemical characterizations are provided in the Methods section at the end and the Supplementary Information ( Supplementary Figs 1,2 and 3 ). Structural studies using X-ray diffraction (XRD) ( Supplementary Fig. 1 ) show that the FeRh layer grows in a highly [001]-oriented manner on the PMN-PT [001] substrate. In the MBE-grown films ( Supplementary Fig. 2 ), in situ reflection high-energy electron diffraction patterns indicate that the FeRh grew epitaxially. In the following discussion, all the measurements were performed on the films grown by sputtering, unless stated otherwise. Magnetic force microscopy In other previous works on FeRh systems, the temperature dependence of magnetic force microscopy (MFM), FM resonance and photoemission electron microscopy have been used to study the dynamics and nucleation of the AFM–FM phase transition [29] , [30] , [31] , [32] . In this work, we use MFM to determine the temperature dependence of the magnetic state of the as-grown (or a virgin) FeRh film. 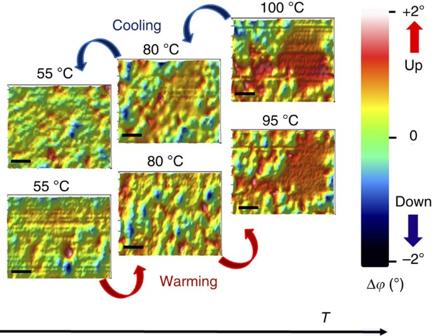Figure 1: MFM images of a FeRh thin film sputtered on a PMN-PT substrate. The false colour indicates the strength and orientation of the magnetic moment (red colour indicates up moment and blue colour down). At low temperature, the non-magnetic signal (Δϕ~0, green colour) of the AFM state dominates and the proportion of magnetic signal from the FM phase increases with temperature. Note that even at 100 °C, which is above the phase-transition temperature, the MFM image shows a coexistence of the AFM phase with the dominant FM phase. Scale bar, 500 nm (black). Figure 1 shows MFM images obtained from the same location on the film at a series of temperatures across the AFM–FM phase transition. The colours represent the relative values of phase shift Δ ϕ measured via dynamic mode MFM and are proportional to the local magnetic field strength and, hence, the proportion of the FM phase. Starting at 55 °C (bottom left in Fig. 1 ) where the AFM phase is dominant, the sample was progressively warmed up to 100 °C, where the FM state is the dominant phase with a small fraction of the AFM phase persisting. On cooling, the fraction of FM phase progressively decreases till 55 °C, at which point the initial AFM-dominant state is restored. These changes in the MFM image and thus the magnetic states are repeatable over different regions of the sample and in multiple samples. Note that the mixed phase is disordered, with no preferred crystallographic orientations for the interfaces between the FM and AFM phases, reminiscent of the behaviour in the CMR manganites [7] , [8] . Figure 1: MFM images of a FeRh thin film sputtered on a PMN-PT substrate. The false colour indicates the strength and orientation of the magnetic moment (red colour indicates up moment and blue colour down). At low temperature, the non-magnetic signal ( Δϕ ~0, green colour) of the AFM state dominates and the proportion of magnetic signal from the FM phase increases with temperature. Note that even at 100 °C, which is above the phase-transition temperature, the MFM image shows a coexistence of the AFM phase with the dominant FM phase. Scale bar, 500 nm (black). Full size image Electrical transport measurement In the following sections, we investigate the transport behaviour. 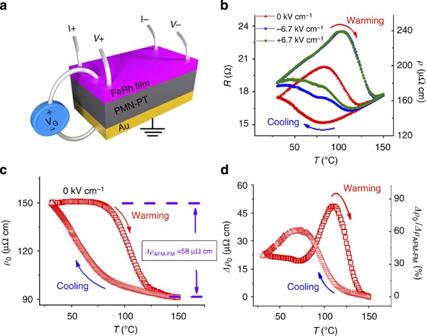Figure 2: Device geometry and electrical transport measurement of FeRh/PMN-PT heterostructure. (a) Schematic of the four-probe device in which theE-field is applied across the FeRh/PMN-PT/Au sandwich structure. (b)ρ−T(orR−T) curve forE-field values of 0 (red), +6.7 kV cm−1(green) and − 6.7 kV cm−1(blue). Hysteresis is clearly visible, with the arrows indicating the warming (red) and cooling (blue) processes. Note that theρ−Tcurve atE=+6.7 kV cm−1and − 6.7 kV cm−1are indistinguishable during the warming. (c)ρ0(E=0) as a function ofTis plotted for the zero-field case. ΔρAFM−FMis defined to be the intrinsic resistivity difference between the AFM and FM phases under no externalE-field and is equal to 58 μΩ cm. (d) The plots of Δρ0(leftyaxis) and Δρ0/ΔρAFM−FM(rightyaxis) versusT. The warming and cooling curves show maximum values in Δρ0/ΔρAFM−FMof ~80% and ~63% at 110 °C and 75 °C, respectively. Figure 2a shows a schematic of the four-probe test structure that was used to carry out the electrical transport measurements. In Fig. 2b , we show the measured resistance R and the corresponding resistivity ρ as a function of temperature T at various electric fields E for a 50-nm-thick FeRh film, both during cooling and warming; the hysteresis is characteristic of a first-order phase transition, consistent with the magnetic property measurements ( Supplementary Figs 4 and 5 ). Figure 2: Device geometry and electrical transport measurement of FeRh/PMN-PT heterostructure. ( a ) Schematic of the four-probe device in which the E -field is applied across the FeRh/PMN-PT/Au sandwich structure. ( b ) ρ−T (or R−T ) curve for E -field values of 0 (red), +6.7 kV cm −1 (green) and − 6.7 kV cm −1 (blue). Hysteresis is clearly visible, with the arrows indicating the warming (red) and cooling (blue) processes. Note that the ρ−T curve at E =+6.7 kV cm −1 and − 6.7 kV cm −1 are indistinguishable during the warming. ( c ) ρ 0 ( E =0) as a function of T is plotted for the zero-field case. Δ ρ AFM−FM is defined to be the intrinsic resistivity difference between the AFM and FM phases under no external E -field and is equal to 58 μΩ cm. ( d ) The plots of Δ ρ 0 (left y axis) and Δ ρ 0 /Δ ρ AFM−FM (right y axis) versus T . The warming and cooling curves show maximum values in Δ ρ 0 /Δ ρ AFM−FM of ~80% and ~63% at 110 °C and 75 °C, respectively. Full size image First, we discuss the zero-field ( E =0) case or a virgin state ( Fig. 2b , red curve). Note that a virgin state is the as-grown FeRh state without any history of E -field applied on the system (no history of pre-poled state). However, regardless of any pre-poled state, the virgin state can easily be recovered by heating up the system up to 150 °C, which is above the Curie temperature (~140 °C) of PMN-PT used in this work, and brought back to room temperature. In this way, we observed strong reproducibility and consistency in resistivity measurement between each thermal cycle at E =0 case, even after the pre-existing poled ( E ≠0) state. We see that the room-temperature ρ of the AFM phase is ~160 μΩ cm, which is comparable to the values in the literature [33] , [34] . The different intrinsic resistivities of the AFM and FM phases, namely Δ ρ AFM−FM , are not apparent in Fig. 2b because of the usual linear increase in metallic resistance with temperature; therefore, we show in Fig. 2c a compensated resistivity ρ 0 ( E =0), which we obtained by removing the linear background increase from the raw data. The linear fitting of the form ρ linear = α ( T − T 0 ), where α is the temperature coefficient and T 0 is a reference temperature, was performed in the AFM state over the 30~70 °C temperature range; this fit was then subtracted from the raw data. We chose T 0 = 30 °C so that the resistivity value after removing the linear background is the same as the raw data at T =30 °C; this offset correction, however, is irrelevant in extracting desired Δ ρ AFM−FM values. In Fig. 2c , Δ ρ AFM−FM is clearly visible and is equal to around 58 μΩ cm. This change in the resistivity is qualitatively consistent with our first-principles density functional calculations ( Supplementary Fig. 6 ), which indicate a large difference in the carrier concentrations at the Fermi level between the FM and AFM phases. Next we discuss the E -field dependence of the transport measurement. In Fig. 2b , we see that both positive (green line) and negative (blue line) E -fields lead to an increase in resistivity over the zero-field case at all temperatures below 140 °C. As the AFM phase has a higher resistivity than the FM phase, this suggests that the E -field increases the fraction of AFM relative to FM phase. Here we attempt to quantify this fractional change between AFM and FM state driven by the E -field. First, we compare the difference in ρ 0 ( E ) values at two fields of E =0 and −6.7 kV cm −1 . Their differences Δ ρ 0 = ρ 0 ( E=− 6.7 kV cm −1 )− ρ 0 ( E=0 ) as a function of T are shown in Fig. 2d (left y axis). Comparing this value with previously calculated Δ ρ AFM−FM , we obtain a ratio Δ ρ 0 /Δ ρ AFM−FM as plotted in Fig. 2d (right y axis). This ratio can be interpreted as the relative fractional change of AFM and FM states with respect to the as-grown states ( E =0) and is an indicator of the efficacy with which the E -field is converting the FM into the AFM phase. Electro-magnetic coupling For further understanding of the magnetic state change in FeRh by an applied E -field, we measured resistivity versus E -field at a fixed temperature (isothermal ρ−E curve) close to the phase transition. In Fig. 3a , we show the relative change in resistivity as function of an applied E -field, defined as Δ ρ/ρ min =[ ρ ( E )− ρ min ]/ ρ min , where ρ min is the minimum resistivity taken at a given isothermal ρ−E curve, for various temperatures near the transition. We term this relative change the ‘giant ER’ (GER) effect. Interestingly, we find a clear hysteresis in Δ ρ/ρ min versus E curves at all the temperatures presented here. In Fig. 3b , we show the maximum values of Δ ρ/ρ min as a function of temperature. Note that these are unusually large for a metallic system, reaching the maximum value of ~8% at 95 °C near the middle of the magnetic phase transition. 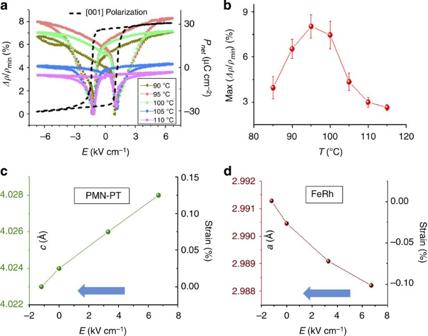Figure 3: The strain-mediated GER effect. (a) Δρ/ρminas a function ofE-field (isothermal curve) for five temperatures between 90 °C and 110 °C. The net polarization along the [001] direction versusE-field of the PMN-PT substrate is overlaid (black-dashed line, rightyaxis). Note the coercivityE-field in the polarization curve is ±1.2 kV °C cm−1. (b) Temperature dependence of the maximum of the ratio Δρ/ρmin,Max(Δρ/ρmin), showing a peak value around 95 °C. To check the reproducibility of GER effect Δρ/ρminversusEcurves were measured repeatedly during a thermal cycling of warming up to 150 °C, cooling down to room temperature, then brought back to the same temperatures where the curves were taken. Remarkably, the data show strong reproducibility during these thermal cycling processes and the error bar in the graph was estimated to account for the small variations inMax(Δρ/ρmin) between the cycles. Lower panels are the lattice constant change (leftyaxes) and the strain (rightyaxes) of PMN-PT (c) and FeRh (d) along their crystalline axes, obtained from XRD measurements within situ E-field application. The maximum compressive IP strain induced in FeRh is 0.1% atE-field of+6.7 kV cm−1. The blue arrows indicate the measurement direction. Figure 3: The strain-mediated GER effect. ( a ) Δ ρ / ρ min as a function of E -field (isothermal curve) for five temperatures between 90 °C and 110 °C. The net polarization along the [001] direction versus E -field of the PMN-PT substrate is overlaid (black-dashed line, right y axis). Note the coercivity E -field in the polarization curve is ±1.2 kV °C cm −1 . ( b ) Temperature dependence of the maximum of the ratio Δ ρ / ρ min , Max (Δ ρ / ρ min ), showing a peak value around 95 °C. To check the reproducibility of GER effect Δ ρ / ρ min versus E curves were measured repeatedly during a thermal cycling of warming up to 150 °C, cooling down to room temperature, then brought back to the same temperatures where the curves were taken. Remarkably, the data show strong reproducibility during these thermal cycling processes and the error bar in the graph was estimated to account for the small variations in Max (Δ ρ / ρ min ) between the cycles. Lower panels are the lattice constant change (left y axes) and the strain (right y axes) of PMN-PT ( c ) and FeRh ( d ) along their crystalline axes, obtained from XRD measurements with in situ E -field application. The maximum compressive IP strain induced in FeRh is 0.1% at E -field of+6.7 kV cm −1 . The blue arrows indicate the measurement direction. Full size image To investigate the electro-magnetic coupling of the FeRh/PMN-PT heterostructure, we measured net polarization P net versus E -field of the PMN-PT along the [001] out-of-plane (OOP) direction (black dashed line in Fig. 3a ). Following a theory of ferroelectrics [35] and a ferroelectric switching model [36] , [37] , a strain can be expressed as a function of P net and vice versa. According to this model, OOP strain in PMN-PT reaches maximum values (tensile strain) when an absolute value of the net polarization | P net | takes its maximum at E =± 6.7 kV cm −1 . On the other hand, the strain reaches zero state when | P net | becomes zero at E =±1.2 kV cm −1 : these values are coercive fields of the PMN-PT polarization curve as shown in Fig. 3a . This further implies that PMN-PT is at its maximum compressive in-plane (IP) strain state at E =± 6.7 kV cm −1 and zero strain state at E =±1.2 kV cm −1 . We observed that the minimum resistivity state of the FeRh film occurs at P net =0, and the maximum resistivity changes occurs at the maximum value of | P net |. Although an induced strain in a ferroelectric results from its net polarization change, the re-alignment of individual ferroelectric domains could also give rise to similar polarization change without inducing significant strain in the material. To rule out the domain re-alignment scenario and therefore validate the direct link between | P net | and strain induced in PMN-PT, we measured PMN-PT lattice constant changes directly using XRD with in-situ E -field application (please note that a larger size of FeRh/PMN-PT sample with the identical growth condition was used for XRD measurement to improve XRD diffraction intensity). The results are shown in Fig. 3c (for the complete XRD spectra, refer to Supplementary Fig. 7 ). Interestingly, PMN-PT shows the maximum OOP lattice constant c =4.028 Å at E=+ 6.7 kV cm −1 and then monotonically decreases to the minimum value of c =4.023 Å as the field is brought down to −1.2 kV cm −1 . The direct measurement of PMN-PT c -values under E -field strongly supports that the polarization switching of PMN-PT does indeed induce the strain modulation rather than re-alignment of small domains within. We further investigated the IP lattice constant a of FeRh as function of E -field and the values are plotted in Fig. 3d . The change in a of FeRh is clearly seen and strongly correlated with the change in PMN-PT c -values. The corresponding strain modulations for both PMN-PT and FeRh are plotted in Fig. 3c,d on the right y axes. Please note that the strains are calculated with respect to the value at E=−1.2 kV cm −1 , where P net =0. In other ferroelectric experiments [26] , [38] , strains are usually calculated with respect to zero E -field value, to account for the pre-poled state of the ferroelectric systems under the study. However, the choice of zero strain state in our work, to be consistent with a theory, does not alter the qualitative conclusion between the strain and resistivity changes of FeRh. With comprehensive observation of the lattice changes on both PMN-PT and FeRh, the net polarization measurement and the hysteresis behaviour in the FeRh/PMN-PT system, we conclude the induced strain to the FeRh/PMN-PT heterostructure by external E -field is responsible for the resistivity modulation of FeRh, presumably altering its magnetic property. Lastly, we demonstrate a rudimentary manifestation of the applicability of such an approach for a potentially low-energy information storage element. In Fig. 4a , we show the hysteresis in Δ ρ/ρ min versus E -field when tested in both bipolar and quasi-bipolar cycling with continuous DC electric field. Then non-volatile logic states were written by applying pulsed-electric field with width of 1 s and amplitude of+1.2 kV cm −1 for the ‘On’ state and −6.7 kV cm −1 for the ‘Off’ state consecutively, as seen in Fig. 4b . The two logic states show strong stability and reproducibility (over the total measurement time of 5 h) and maintain clearly differentiated resistivity values in each state. 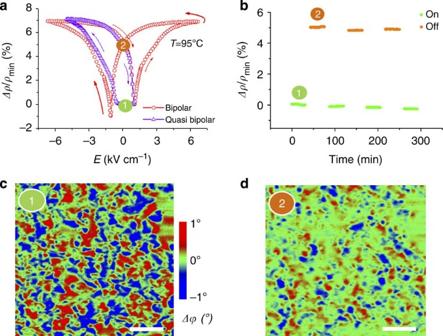Figure 4: Potential application to ferroelectric RAM memory device and magnetic phase modulation by electric field. (a) Δρ/ρminversusE-field in bipolar and quasi-bipolar curves. Continuous DCE-fields were used in the plot and the arrows indicate the direction of theE-field sweep. (b) The plot shows Δρ/ρminas a function of time in the ‘On’ state (lowerρstate, 1) and ‘OFF’ state (higherρstate, 2). Two different logic states were written by pulsedE-fields with the amplitudes of +1.2 kV cm−1(On state, 1) and −6.7 kV cm−1(Off state, 2) consecutively for each state. Each state lasts for 30 min and the On/Off states were stable and reproducible over seven consecutive sequences. Two MFM images were taken at these two states with On-state (c) and Off-state (d) reproduced by the same pulsedE-fields. The vertical colour scale bar (in the middle) shows the phase shift Δϕin MFM and proportional to the local magnetic moment strength. Scale bar, 1 μm (white). Figure 4: Potential application to ferroelectric RAM memory device and magnetic phase modulation by electric field. ( a ) Δ ρ / ρ min versus E -field in bipolar and quasi-bipolar curves. Continuous DC E -fields were used in the plot and the arrows indicate the direction of the E -field sweep. ( b ) The plot shows Δ ρ / ρ min as a function of time in the ‘On’ state (lower ρ state, 1) and ‘OFF’ state (higher ρ state, 2). Two different logic states were written by pulsed E -fields with the amplitudes of +1.2 kV cm −1 (On state, 1) and −6.7 kV cm −1 (Off state, 2) consecutively for each state. Each state lasts for 30 min and the On/Off states were stable and reproducible over seven consecutive sequences. Two MFM images were taken at these two states with On-state ( c ) and Off-state ( d ) reproduced by the same pulsed E -fields. The vertical colour scale bar (in the middle) shows the phase shift Δ ϕ in MFM and proportional to the local magnetic moment strength. Scale bar, 1 μm (white). Full size image To understand the origin of resistivity modulation by E -field, two MFM images of FeRh were taken at the ‘On’ ( Fig. 4c ) and ‘Off’ states ( Fig. 4d ). The images show magnetic phase changes between these two logic states, with ‘On’ state (lower resistivity) showing stronger magnetic signal and the ‘Off’ state (higher resistivity) showing suppressed magnetic signal. The phase shift Δ ϕ indicates the strength of local magnetic moments, and therefore green colours correspond to zero (or very weak) magnetic moment in the region. In both images, we observed a mixture of AFM (green) and FM (blue and red), and the difference in these two images shows that the role of the strain induce by E -field is to convert the relative ratio between them. Our first-principles density functional calculations ( Supplementary Fig. 6 ) indicate negligible changes in the electronic and magnetic structure of either the FM or AFM phase at the limit of two extreme cases: 0.1% tensile and compressive strain. The calculation suggests that the role of the strain is to convert between the FM and AFM phases, resulting in the large change in the resistivity observed in this experiment. Combined with the MFM observation and the density functional theory calculation, the resistivity modulation of FeRh is a direct consequence of the magnetic phase variation (or the AFM to FM ratio changes), mediated via strain modulation of ferroelectric substrate, influenced by external E -field. In summary, we have reported the GER effect in FeRh/PMN-PT heterostructures, via the strain control of a ferroelectric substrate. 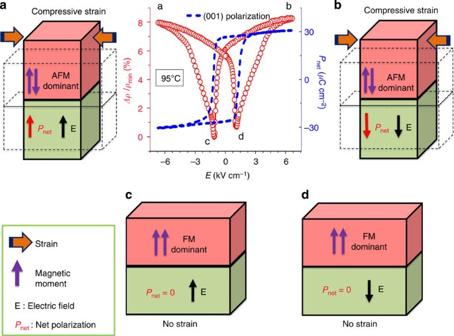Figure 5: Schematics for the reversible resistivity modulation by anE-field in a FeRh/PMN-PT heterostructure. (a,b) The compressive IP strain state promotes the AFM-dominant state leading to a higher resistivity state with a Δρ/ρminvalue up to 8%. (c,d) No-strain state, which promotes an FM-dominant state of FeRh, and Δρ/ρmintakes its minimum value. The inset in the middle are plots of Δρ/ρmin(red, leftyaxis) andPnet(blue, rightyaxis) as a function ofE-field. Figure 5 summarizes the schematic diagram of the strain dynamics on the FeRh/PMN-PT system whose resistivity can reversibly be controlled by an external E -field. Comprehensive studies of MFM and X-ray diffractometer combined with resistivity measurements reveal that the compressive IP strain on FeRh drives the system into more AFM-dominated state, and therefore a higher resistivity state is achieved ( Fig. 5a,b ). On the other hand, when the system relaxes back to no-strain state, FM state is preferred ( Fig. 5c,d ), leading to a lower resistivity state. We showed that the origin of the resistivity change is the conversion between the coexisting FM and AFM phases of FeRh, which have different volumes and conductivities accompanying the different magnetic orderings. The strain-mediated resistivity change is large for a metallic/ferroelectric heterostructure system at E -fields of the order of 4~6 kV cm −1 , rendering the behaviour potentially technologically relevant. This sensitivity is a consequence of the fact that the FM and AFM phases are relatively close in energy near the transition temperature [24] and thus can be interconverted from one to the other by simply straining the lattice parameter of the system. Artificially engineered heterostructures such as spin valves or tunnel junction devices may enhance the control of resistance modulation and therefore make the GER effect found in this work more attractive for applications. Figure 5: Schematics for the reversible resistivity modulation by an E -field in a FeRh/PMN-PT heterostructure. ( a , b ) The compressive IP strain state promotes the AFM-dominant state leading to a higher resistivity state with a Δ ρ / ρ min value up to 8%. ( c , d ) No-strain state, which promotes an FM-dominant state of FeRh, and Δ ρ / ρ min takes its minimum value. The inset in the middle are plots of Δ ρ / ρ min (red, left y axis) and P net (blue, right y axis) as a function of E -field. Full size image Film growth and characterization FeRh films were fabricated by both DC sputtering and MBE techniques. For the sputtering deposition, (001)-oriented PMN-PT substrates (1-μm-thick Au layer was coated on the back side as bottom electrodes as in Fig. 2a ) were heated up to 375 °C at the rate of 20 °C min −1 in a base pressure of 10 −8 Torr. Subsequently, a small amount of Ar gas was introduced into the chamber, maintaining the total pressure of 3.0 mTorr. The FeRh films were then grown from a stoichiometric Fe 0.5 Rh 0.5 target. After the deposition, films were heated up to 500 °C at 10 °C min −1 in vacuum and annealed for 1 h and subsequently cooled to room temperature at 10 °C min −1 . The deposition rate was 1.75 nm min −1 , determined by X-ray reflectivity measurements. MBE films were grown in a Veeco Gen10 MBE chamber with a chamber background pressure of ~8 × 10 −9 Torr. The FeRh films were deposited at a substrate temperature of 420 °C. The orientation and phase purity of the growth of the epitaxial FeRh films was monitored in situ via reflection high-energy electron diffraction. Following the deposition, the films were annealed at the same temperature for 30 min. XRD spectra with in situ E -fields were collected in a PANalytical X’Pert PRO diffractometer combined with a Keithley 2410 voltage source meter. Chemical analysis The chemical composition of the FeRh films was analysed by nano-Auger Electron Spectroscopy conducted in ultra-high vacuum (base pressure ~10 −10 mbar) using a field-emission electron source whose spot size was focused below a diameter of 10 nm and a multi-channel hemispherical energy analyser. After removal of the surface oxide layer by gentle Ar ion milling, the chemical stoichiometry of FeRh films was estimated to be Fe 0.44 Rh 0.56 , using primary Rh MNN and Fe LMM Auger peaks. This value is within the composition range of the FeRh α ′-phase showing the AFM–FM transition. Magnetic force microscopy MFM measurements were acquired using a non-contact tapping mode and a dynamic lift variation with a lift height of 30 nm. This was repeated at various temperatures using a Veeco Nanoscope with the temperature control capability up to 150 °C. Electrical transport measurement Resistance measurements from 30 to 150 °C were carried out in a typical four-probe stage setup using the van der Pauw geometry with an external current source (Keithley-6220) and voltage meter (Keithley-2182). DC electric fields of up to±6.7 kV cm −1 were provide by a Keithley-6517B voltage source and were applied between the top FeRh film and the bottom Au electrode on the underside of the PMN-PT substrate with the bottom electrode grounded ( Fig. 2a ). For the pulsed electric field used for generating the two logic states in Fig. 4b , a wave-form generator (Agilent 33250A) with a voltage amplifier was used. Magnetic property measurements Magnetization measurements were carried out in a superconducting quantum interference device magnetometer by Quantum Design with a maximum temperature capability of 400 K. Density functional theory calculations We computed the electronic densities of states of the AFM and FM phase of FeRh in the CsCl structure for two extreme cases: 0.1% tensile and compressive strain along the [100] IP direction, using Vienna ab initio simulation package [39] , [40] , [41] , [42] with the Perdew–Burke–Ernzerhof exchange correlation functional [43] , and projector augmented wave potentials [44] , [45] with Fe (4 s , 3 d , 3 p ) and Rh (5 s , 4 d , 4 p ) valence electrons. The plane-wave cutoff was 550 eV and reciprocal space was sampled with 19 × 19 × 19 and 11 × 11 × 11 Γ-centred meshes for the FM and AFM (2 × 2 × 2 supercell) phases, respectively. How to cite this article: Lee, Y. et al . Large resistivity modulation in mixed-phase metallic systems. Nat. Commun. 6:5959 doi: 10.1038/ncomms6959 (2015).